G-protein stimulatory subunit alpha and Gq/11α G-proteins are both required to maintain quiescent stem-like chondrocytes Round chondrocytes in the resting zone of the growth plate provide precursors for columnar chondrocytes and have stem-like properties. Here we demonstrate that these stem-like chondrocytes undergo apoptosis in the absence of the receptor (PPR) for parathyroid hormone-related protein. We examine the possible roles of heterotrimeric G-proteins activated by the PPR. Inactivation of the G-protein stimulatory α-subunit (G s α) leads to accelerated differentiation of columnar chondrocytes, as seen in the PPR knockout, but a remnant of growth cartilage remains, in contrast to disappearance of the growth cartilage in the PPR knockout. Stem-like chondrocytes lose their quiescence and proliferate upon G s α ablation. Inactivation of G s α in mice with a mutant PPR that cannot activate G proteins, Gq and G11, leads to a PPR knockout-like phenotype. Thus, G s α is the major mediator of the anti-differentiation action of the PPR, while activation of both G s α and Gq/11α is required for quiescence of stem-like chondrocytes. Postnatal linear growth of long bones of mammalian limbs occurs at the growth plate. The growth plate consists of three distinct layers of chondrocytes, called resting (also called stem-like, reserve or round chondrocytes), proliferative (also called flat or columnar chondrocytes) and hypertrophic chondrocytes. Chondrocytes located in the resting zone, which provide precursors for the underlying columnar chondrocytes, have stem-like properties. This role was first proposed by Kember, based on pulse-chase H 3 -thymidine labelling experiments in which he delineated this slowly dividing cell population and demonstrated that progeny of these cells became columnar chondrocytes [1] , [2] . Furthermore, the resting zone is able to reconstitute the entire growth plate upon surgical removal of the columnar and hypertrophic zones [3] . However, the mechanisms regulating the activity of these cells are unknown. After stem-like chondrocytes leave their quiescent stage, they become flat and form a layer of rapidly dividing cells organized in orderly columns. These chondrocytes then stop proliferating, hypertrophy, mineralize their matrix and die by apoptosis. Thereafter, the mineralized scaffold is replaced by newly invading osteoclasts, osteoblasts and blood vessels. This process of bone growth is referred to as endochondral ossification [4] . Parathyroid hormone-related protein (PTHrP) and Indian hedgehog (Ihh) form a negative feedback loop that controls the differentiation of chondrocytes in the fetal growth plate [5] . Actions of PTHrP are mediated through the parathyroid hormone (PTH)/PTHrP receptor (PPR), a G protein-coupled receptor that can activate multiple heterotrimeric G proteins. This receptor activates both the stimulatory G protein α-subunit (G s a) (that activates adenylyl cyclase and the protein kinase A (PKA) pathway) and the closely related G q α and G 11 α G-proteins (that activate phospholipase C and the downstream PKC/Ca ++ pathway) [6] . Further, in cultured osteoblastic cells, the PPR can also activate Gα12/1 3G-proteins [7] . The roles of G s α and G q/11 α in mediating the actions of PTHrP in the fetal growth plate have been studied through genetic manipulation in mice. Knockout of either PPR or G s α in fetal chondrocytes accelerates chondrocyte hypertrophy [8] . In contrast, mice with a PPR that activates G s α normally but cannot activate G q/11 α exhibit a delay in hypertrophy in fetal life [9] . We have shown that postnatal ablation of the PPR in the epiphyseal growth plate leads to abrupt disappearance (fusion) of the growth plate in mice [10] . Ablation of the PPR was associated with increased rates of apoptosis in the resting zone. Here we have inactivated G-protein stimulatory subunit alpha (G s α) in the postnatal growth plate and observed neither fusion of the growth plate nor elevated apoptosis in the resting zone. We found altered behaviour of stem-like chondrocytes and found that activation of G s α together with G q α/G 11 α is required for stem-like chondrocytes to remain quiescent. Ablation of G s α leads to slowed growth and remnant formation We used a tamoxifen-dependent cre recombinase (CreERt) driven by the collagen II (Col2) promoter to ablate G s α through matings with mice in which exon 1 of G s α is flanked by lox sites [11] . Inactivation of G s α in the postnatal growth plate induced marked growth retardation, including significant decrease in body weight and shortening of both the axial and appendicular skeleton ( Fig. 1a,b , Supplementary Fig. 1a,b ). There was no effect of the Col2-CreERt transgene alone on bone growth and growth plate morphology as it was shown early [10] and can also be seen below. Activity of Cre in the postnatal growth plate upon tamoxifen administration was verified utilizing breeding with Rosa 26 reporter mice and X-gal staining ( Fig. 1c ; 95±1% X-gal positive cells in the resting zone, 98±1% in the proliferative and 59±8% in the hypertrophic zone, 5 days after tamoxifen administration, n =3, data presented as mean±s.e.m. here and everywhere below). Expression of G s α mRNA was observed mainly in prehypertrophic (Ihh-expressing) and hypertrophic (Ihh and Collagen type X-expressing) chondrocytes ( Fig. 1d ). Decreased expression of G s α mRNA ( Fig. 1d ) and recombination of GNAS1 DNA ( Supplementary Fig. 1c ) in the growth plate chondrocytes were observed upon tamoxifen administration. 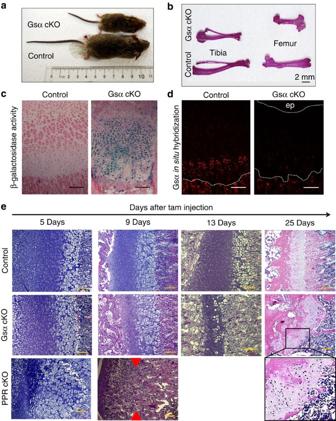Figure 1: Postnatal ablation of Gsα in chondrocytes leads to severe growth retardation and cartilage remnant formation. Representative pictures of control (Gsα fl/fl) and Gsα cKO (Col2-CreERt; Gsα fl/fl) (a) mice and (b) their long bones stained with Alizarin Red 1 month after tamoxifen administration. (c) Cre activity in the growth plate was monitored with a Rosa 26 reporter (Rosa). Control (Gsα fl/fl; Rosa/+) and Gsα cKO (Col2-CreERt; Gsα fl/fl; Rosa/+) mice were injected with tamoxifen, and x-gal staining was performed 5 days later. Sections were counterstained with Eosin. (d) Levels of Gsα mRNA were assayed 9 days after tamoxifen administration byin situhybridization. Dashed lines depict the growth plate. ep, epiphyseal bone. (e) Time course of changes in the tibial growth plate upon ablation of Gsα or PTH receptor (PPR), which was performed utilizing an identical protocol and the same Col2-CreERt strain. Accelerated differentiation (day 5) followed by fusion of the growth plate (day 9, depicted by red arrowheads) was observed upon PPR ablation. Narrowing of the growth plate (day 9), followed by disorganization (day 13) and cartilage remnant formation (day 25) was observed upon Gsα ablation. In all experiments, tamoxifen was injected i.p. at 3 days of age. Scale bar, 100 μm (c–e). Figure 1: Postnatal ablation of G s α in chondrocytes leads to severe growth retardation and cartilage remnant formation. Representative pictures of control (G s α fl/fl) and G s α cKO (Col2-CreERt; G s α fl/fl) ( a ) mice and ( b ) their long bones stained with Alizarin Red 1 month after tamoxifen administration. ( c ) Cre activity in the growth plate was monitored with a Rosa 26 reporter (Rosa). Control (G s α fl/fl; Rosa/+) and G s α cKO (Col2-CreERt; G s α fl/fl; Rosa/+) mice were injected with tamoxifen, and x-gal staining was performed 5 days later. Sections were counterstained with Eosin. ( d ) Levels of G s α mRNA were assayed 9 days after tamoxifen administration by in situ hybridization. Dashed lines depict the growth plate. ep, epiphyseal bone. ( e ) Time course of changes in the tibial growth plate upon ablation of G s α or PTH receptor (PPR), which was performed utilizing an identical protocol and the same Col2-CreERt strain. Accelerated differentiation (day 5) followed by fusion of the growth plate (day 9, depicted by red arrowheads) was observed upon PPR ablation. Narrowing of the growth plate (day 9), followed by disorganization (day 13) and cartilage remnant formation (day 25) was observed upon G s α ablation. In all experiments, tamoxifen was injected i.p. at 3 days of age. Scale bar, 100 μm ( c – e ). Full size image Next, we followed time-dependent changes in the growth plate upon G s α ablation. We did not observe any significant differences in the growth plate phenotype of Col2-CreERt;G s α fl/fl (G s α cKO) mice 5 days after tamoxifen administration ( Fig. 1e ; height of the growth plate 1,063±14 in control versus 1,030±21 μm in G s α cKO mice, P =0.26 by t -test; height of the hypertrophic zone 191±7 in control versus 207±8 μm in G s α cKO mice, P =0.17 by t -test, n =4, data presented as mean±s.e.m. here and everywhere below). This is a time period sufficient to induce marked acceleration of hypertrophy upon ablation of the PPR (Col2-CreERt;PPR fl/fl (PPR cKO) mice) ( Fig. 1e and see ref. 10 ); height of the growth plate 997±30 versus 1,063±14 μm in control ( P =0.3 by t -test, n =3) and height of the hypertrophic zone 431±11 versus 191±7 μm in control; P <0.001 by t -test, n =3). Nine days after administration of tamoxifen, a time point at which the PPR cKO mice already had fused their growth plates ( Fig. 1e , see also ref. 10 ), the growth plate height was reduced in G s α cKO mice (333±20 versus 540±20 μm in control, P <0.001 by t -test, n =8). This reduction was associated with reduction of the height of the flat cell layer ( Supplementary Fig. 1d ). The height of the hypertrophic zone was not significantly affected by G s α ablation ( Supplementary Fig. 1d ; P =0.32 by t -test, n =8), whereas the height of the terminally hypertrophic chondrocytes (marked by a domain of osteopontin expression) was decreased (17.2±1.2 versus 22.1±0.6 μm in control, n =5, P <0.01 by t -test) and number of hypertrophic chondrocytes per column was increased (13.3±0.4 versus 8.6±0.6 in control, n =8, P <0.001 by t -test). Thirteen days after tamoxifen injection, the growth plate of G s α cKO mice further shortened and became disorganized, with flat and hypertrophic cells mixed together ( Fig. 1e ). One month after G s α ablation, the growth plate of G s α cKO mice transformed into a disorganized structure, which we call the cartilage remnant ( Fig. 1e , see also examples throughout the figures). G s α ablation accelerates only chondrocyte differentiation The changes in cell number in each of the chondrocyte layers may be caused by changes in cell proliferation, rates of cell differentiation or changes in apoptosis. We evaluated these processes for 3 time-points after tamoxifen administration. Five days after tamoxifen injection, chondrocyte proliferation was not significantly affected upon G s α ablation (20±3% in control versus 17±2% in G s α cKO mice, n =4, P =0.45 by t -test (calculated as a number of BrdU-positive columnar chondrocytes divided by the total number of columnar chondrocytes in the area in which BrdU-positive cells were detected)). In contrast, at this time point, ablation of the PPR decreased chondrocyte proliferation (20±1% in control versus 8±0.6% in PPR cKO, n =3, P <0.01 by t -test; see also Supplementary Fig. 1e ). At this time point, an increased number of TUNEL-positive cells was observed in the resting zone of PPR cKO mice (1.1±0.2% in control versus 3.9±0.3% in PPR cKO mice, P <0.01 by t -test, n =3). Below, we will clarify that this increase in TUNEL-positive cells largely represents death of stem-like chondrocytes. Nine days after tamoxifen administration, reduction in the flat cell layer in the G s α cKO mice ( Supplementary Fig. 1d ) was not accompanied by reduction in the rate of proliferation. Instead, proliferation was slightly albeit not significantly elevated (17±1% BrdU-positive cells (pink) in control versus 21±3% in G s α cKO mice, n =3, P =0.24 by t -test, see also Fig. 2a and Supplementary Fig. 2c ). This observation was further supported by a slight increase in the number of Ki67-positive cells (141±3 cells per mm 2 in control versus 179±5 cells per mm 2 in G s α cKO mice, n =3, P =0.08 by t -test, Supplementary Fig. 2a ). Interestingly, flat chondrocytes that do not incorporate BrdU (post-mitotic flat chondrocytes) were not observed in G s α cKO mice, though they were prominent in the WT mice (blue nuclei depicted in Fig. 2a ). These cells were not eliminated by apoptosis since elevated number of TUNEL-positive cells was observed only at the chondro–osseous junction in the G s α cKO mice (flat zone (%): 1.5±0.2 versus 1.8±0.4 for control and G s α cKO mice, respectively, P =0.53 by t -test, n =5; chondro–osseous junction (cells per mm of the junction): 8.1±1.0 versus 28.1±1.7 for control and G s α cKO mice, respectively, P <0.001 by t -test, n =5; Fig. 2b ). These data, combined with the increased number of hypertrophic chondrocytes per column in the G s α cKO mice (see above), suggest that ablation of G s α accelerates differentiation of flat chondrocytes into hypertrophic chondrocytes. Indeed, domains of expression of both Collagen X mRNA (Col X) and Indian hedgehog mRNA (Ihh), markers of chondrocyte differentiation, were clearly expanded in G s α cKO mice (height of ColX domain 96±9 in control versus 146±13 μm in G s α cKO mice ( P <0.05 by t -test, n =3) and height of Ihh domain 97±2 in control versus 188±31 μm G s α cKO mice ( P <0.05 by t -test, n =3); see also Fig. 2c,d ). The domain of osteopontin-expressing, terminally differentiated chondrocytes was not expanded (63±6 versus 60±9 μm, P =0.85 by t -test, n =3, see also Supplementary Fig. 2b ). 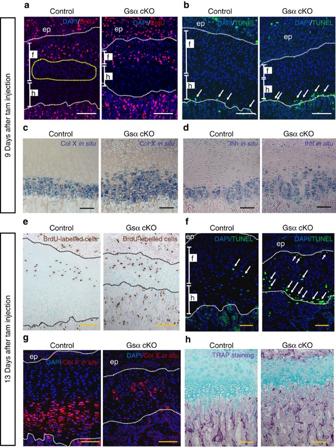Figure 2: Gsα ablation does not affect chondrocyte proliferation but accelerates differentiation and apoptosis. Tamoxifen was administrated at 3 days of age and growth plates were analysed 9 (a–d) and 13 (e–h) days later. Chondrocyte proliferation was not affected (a, pink cells, BrdU labelling for 2 hours), but post-mitotic flat cells were missed in Gsα cKO mice (depicted by yellow dotted line). Increase in the TUNEL-positive cells was observed at the chondro–osseous junction in Gsα cKO mice as compared with controls (b, green cells). At the same time, elevated numbers of cells expressing collagen type X mRNA (c) and Indian Hedgehog mRNA (d) were observed in Gsα cKO mice as compared with controls. (e) BrdU-positive chondrocytes (brown) were observed throughout the growth plate of Gsα cKO mice 13 days after gene ablation. Sections were counterstained with Eosin (pink) and Alcian Blue (blue). (f) TUNEL-positive cells (green) were detected mainly at the metaphyseal side of the growth plate but also at the epiphyseal side and in the middle of the growth plate 13 days after gene ablation. (g) Collagen type X mRNA (pink) was detected in the middle of the growth plate in Gsα cKO mice at this time point. (h) There was no increase in osteoclast activity in Gsα cKO mice as detected by TRAP staining. Dotted lines depict growth plates. f=flat cell layer; h=hypertrophic layer. Arrows show typical apoptotic chondrocytes. ep=epiphyseal bone. Scale bars, 100 μm. Figure 2: G s α ablation does not affect chondrocyte proliferation but accelerates differentiation and apoptosis. Tamoxifen was administrated at 3 days of age and growth plates were analysed 9 ( a – d ) and 13 ( e – h ) days later. Chondrocyte proliferation was not affected ( a , pink cells, BrdU labelling for 2 hours), but post-mitotic flat cells were missed in G s α cKO mice (depicted by yellow dotted line). Increase in the TUNEL-positive cells was observed at the chondro–osseous junction in G s α cKO mice as compared with controls ( b , green cells). At the same time, elevated numbers of cells expressing collagen type X mRNA ( c ) and Indian Hedgehog mRNA ( d ) were observed in G s α cKO mice as compared with controls. ( e ) BrdU-positive chondrocytes (brown) were observed throughout the growth plate of G s α cKO mice 13 days after gene ablation. Sections were counterstained with Eosin (pink) and Alcian Blue (blue). ( f ) TUNEL-positive cells (green) were detected mainly at the metaphyseal side of the growth plate but also at the epiphyseal side and in the middle of the growth plate 13 days after gene ablation. ( g ) Collagen type X mRNA (pink) was detected in the middle of the growth plate in G s α cKO mice at this time point. ( h ) There was no increase in osteoclast activity in G s α cKO mice as detected by TRAP staining. Dotted lines depict growth plates. f=flat cell layer; h=hypertrophic layer. Arrows show typical apoptotic chondrocytes. ep=epiphyseal bone. Scale bars, 100 μm. Full size image Proliferation remained elevated 13 days after G s α ablation (14±2% of BrdU-positive cells in control versus 22±1% in G s α cKO mice ( P <0.001 by t -test, n =4; calculated as a number of BrdU-positive chondrocytes divided by the total number of chondrocytes in the area in which BrdU-positive cells were detected), see also Fig. 2e ). At this time point the growth plate had become disorganized ( Fig. 1e ). Apoptotic cells were observed not only at the chondro–osseous junction but also throughout the growth plate ( Fig. 2f ). Cells expressing collagen type X mRNA were observed in all the different zones of the growth plate of G s α cKO mice ( Fig. 2g ). The interface between the end of the growth plate and the primary spongiosa was not obviously disrupted: the terminal layer of hypertrophic chondrocytes was of normal length, as indicated by normal osteopontin mRNA levels in the late hypertrophic layer ( Supplementary Fig. 2b ), and the number of osteoclasts in the primary spongiosa was not affected ( Fig. 2h ). We next characterized cellular and molecular properties of the cartilage remnant to identify possible reasons for the existence of this unusual structure. First, we found that the remnant remained in the bone for at least several months ( Fig. 3a ) and thereafter focused all the following characterization at 4 weeks of age; a time point right after the remnant is fully formed. No proliferative cells were observed in the cartilage remnant ( Fig. 3b ). The remnant was Alcian blue positive ( Fig. 3b ), whereas Collagen X mRNA was not detected ( Fig. 3c ). Some cells in the remnant expressed Ihh mRNA, a gene normally expressed by prehypertrophic chondrocytes ( Fig. 3d ). This observation suggests that chondrocytes in the remnant may be in post-mitotic and pre-hypertrophic stages of differentiation. To demonstrate the robustness of the remnant phenotype, we performed a series of control experiments. G s α mRNA ( Fig. 3e ) as well as G s α protein (demonstrated in the double G s α plus XLαs mutants due to antibody cross-reactivity between G s α and XLαs, see below) was not detected, whereas DNA recombination of the Gnas gene ( Fig. 3g ) and β-gal activity, indicating action of cre recombinase ( Fig. 3f ), were observed in the remnant. Higher doses or longer duration of tamoxifen treatment did not facilitate the growth plate disappearance in G s α cKO mice ( Supplementary Fig. 3a ). Formation of a cartilage remnant upon G s α ablation was observed in mice of both C57/BL6 and CD-1 backgrounds (see Methods section for details). Breeding to ablate G s α and one or two copies of the PPR gene revealed that within the same litter, mice without the PPR fused their growth plates even in the absence of G s α ( Supplementary Fig. 3b ). In contrast, mice without G s α form the growth plate remnant even in the presence of only one allele of the PPR gene ( Supplementary Fig. 3c ). Notice that there was no effect of the Col2-CreERt transgene alone on bone growth and growth plate morphology ( Supplementary Fig. 3b,c ). Thus, we conclude that ablation of the G s α gene in postnatal mice leads to growth retardation, accelerated chondrocyte proliferation and differentiation, and disorganization of the growth plate with subsequent formation of a cartilage remnant. 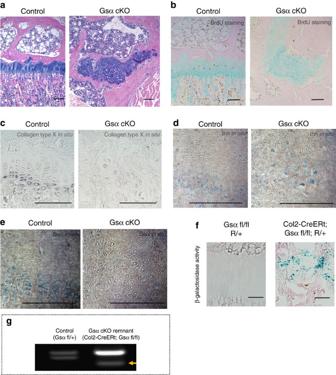Figure 3: Characterization of the cartilage remnant. Tamoxifen was injected at 3 days of age and growth plates were analysed 3 (a) or 1 month later (b–g). (a) The remnant remained in the bone 3 months after tamoxifen injection. (b) BrdU incorporation was detected in the growth plate of control (Gsα fl/fl) mice, but not in the remnant of Gsα cKO mice (BrdU injected 4 and 24 h before death). Sections were counterstained with Eosin (bone, pink) and Alcian Blue (cartilage, blue). (c) Collagen X mRNA was not detected in the remnant. (d) Some remnant cells were positive for Ihh mRNA, marker for prehypertrophic chondrocytes. (e) Gsα mRNA was not detected in the remnant of Gsα cKO mice, while prehypertrophic chondrocytes were positive in control mice. (f) β-galactosidase activity was detected in the remnant of Gsα cKO; Rosa reporter mice. X-gal staining was performed on non-fixed, non-decalcified frozen sections and counterstained with eosin. R=Rosa26. (g) Recombination ofGNAS1gene was detected in DNA isolated from the microdissected remnant (yellow arrowhead,g). The non-recombinant band in Gsα cKO mice is prominent, presumably due to contamination with Cre-negative surrounding tissue during microdissection. The upper band in the heterozygous control corresponds to the floxed allele and the lower band to the wild-type allele. Scale bars, 100 μm. Figure 3: Characterization of the cartilage remnant. Tamoxifen was injected at 3 days of age and growth plates were analysed 3 ( a ) or 1 month later ( b – g ). ( a ) The remnant remained in the bone 3 months after tamoxifen injection. ( b ) BrdU incorporation was detected in the growth plate of control (G s α fl/fl) mice, but not in the remnant of G s α cKO mice (BrdU injected 4 and 24 h before death). Sections were counterstained with Eosin (bone, pink) and Alcian Blue (cartilage, blue). ( c ) Collagen X mRNA was not detected in the remnant. ( d ) Some remnant cells were positive for Ihh mRNA, marker for prehypertrophic chondrocytes. ( e ) G s α mRNA was not detected in the remnant of G s α cKO mice, while prehypertrophic chondrocytes were positive in control mice. ( f ) β-galactosidase activity was detected in the remnant of G s α cKO; Rosa reporter mice. X-gal staining was performed on non-fixed, non-decalcified frozen sections and counterstained with eosin. R=Rosa26. ( g ) Recombination of GNAS1 gene was detected in DNA isolated from the microdissected remnant (yellow arrowhead, g ). The non-recombinant band in G s α cKO mice is prominent, presumably due to contamination with Cre-negative surrounding tissue during microdissection. The upper band in the heterozygous control corresponds to the floxed allele and the lower band to the wild-type allele. Scale bars, 100 μm. Full size image Further characterization revealed that levels of Mef2c, a transcription factor needed for chondrocyte hypertrophy [12] , were decreased in the remnant, although some positive cells were observed ( Fig. 4a ). Signalling by bone morphogenic proteins (BMPs) can facilitate the production of hypertrophic chondrocytes [13] , [14] . We found that the activity of BMP signalling, assessed by the levels of phosphorylated SMAD-1/5, was also decreased in the remnant ( Fig. 4b ). Further, only a few Sox9-positive cells were detected in the remnant ( Fig. 4c ). These findings suggest widespread disruption of paracrine signalling and transcription factor expression in cells of the remnant. 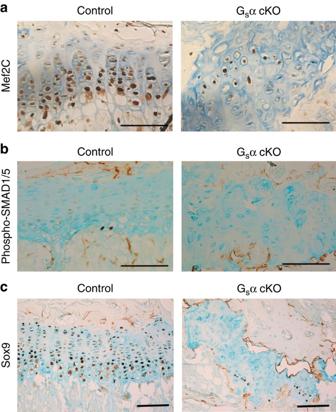Figure 4: Further molecular characterization of the cartilage remnant. Tamoxifen was injected at 3 days of age and growth plates were analysed 1 month later. (a) Mef2C protein was detected immunohistochemically in prehypertrophic and hypertrophic chondrocytes in control mice; a few positive cells were also detected in the cartilage remnant of Gsα cKO mice. (b) phospho-SMAD1/5 was detected immunohistochemically in prehypertrophic and columnar chondrocytes in control mice but not in the remnant. (c) In control mice, Sox9 protein was detected throughout the growth plate. The most intense signal was found in prehypertrophic chondrocytes, whereas only a few cells were positive for Sox9 in the remnant. Scale bars, 100 μm. Figure 4: Further molecular characterization of the cartilage remnant. Tamoxifen was injected at 3 days of age and growth plates were analysed 1 month later. ( a ) Mef2C protein was detected immunohistochemically in prehypertrophic and hypertrophic chondrocytes in control mice; a few positive cells were also detected in the cartilage remnant of G s α cKO mice. ( b ) phospho-SMAD1/5 was detected immunohistochemically in prehypertrophic and columnar chondrocytes in control mice but not in the remnant. ( c ) In control mice, Sox9 protein was detected throughout the growth plate. The most intense signal was found in prehypertrophic chondrocytes, whereas only a few cells were positive for Sox9 in the remnant. Scale bars, 100 μm. Full size image Ablation of G s α forces stem-like chondrocytes to proliferate We next hypothesized that the striking differences in chondrocyte proliferation between the PPR and G s α cKO mice (see Supplementary Fig. 2c ) might be associated with altered behaviour of so-called ‘reserve’ cells (also called ‘round’ cells or stem-like chondrocytes) located at the top of the growth plate as well. To test this hypothesis, we labelled stem-like chondrocytes with multiple BrdU injections followed by a chase period to identify slowly replicating stem-like chondrocytes ( Fig. 5a,b ). One month later, BrdU-positive stem-like chondrocytes were detected at the top of the growth plate in control mice, whereas BrdU-positive cells were absent in the remnant of G s α cKO mice ( Fig. 5c ). Thus, slowly proliferating chondrocytes did not persist in the remnant. 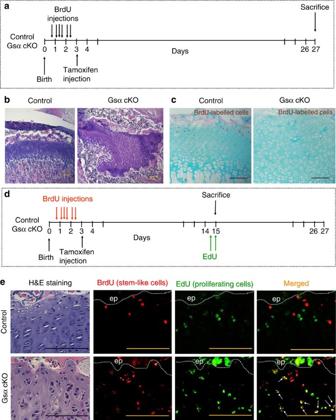Figure 5: Chondrocytes of reserve zone are recruited into proliferation in Gsα cKO mice. (a) Protocol for BrdU labelling of reserve zone cells (stem-like chondrocytes). (b) Representative images of the growth plates of control (Gsα fl/fl) and Gsα cKO (Col2-CreERt; Gsα fl/fl) mice shown ina,c. Sections are stained with H&E. (c) BrdU-detection revealed BrdU-positive stem-like chondrocytes in control, but not in Gsα cKO growth plates. Sections were counterstained with eosin (bone, pink) and Alcian Blue (cartilage, blue). (d) Modified protocol for BrdU labelling of stem-like chondrocytes aiming to detect stem-like cell proliferation. Mice were labelled with BrdU exactly as ina, but were killed earlier and were labelled with EdU 4 and 20 h before death. (e) Sections from control (Gsα fl/fl) and Gsα cKO (Col2-CreERt; Gsα fl/fl) mice treated as shown indwere stained with both BrdU and EdU. Double BrdU- and EdU-labelled cells (arrows) were observed in Gsα cKO mice but almost never in control mice. ep=epiphyseal bone. Scale bars, 100 μm. Figure 5: Chondrocytes of reserve zone are recruited into proliferation in G s α cKO mice. ( a ) Protocol for BrdU labelling of reserve zone cells (stem-like chondrocytes). ( b ) Representative images of the growth plates of control (G s α fl/fl) and G s α cKO (Col2-CreERt; G s α fl/fl) mice shown in a , c . Sections are stained with H&E. ( c ) BrdU-detection revealed BrdU-positive stem-like chondrocytes in control, but not in G s α cKO growth plates. Sections were counterstained with eosin (bone, pink) and Alcian Blue (cartilage, blue). ( d ) Modified protocol for BrdU labelling of stem-like chondrocytes aiming to detect stem-like cell proliferation. Mice were labelled with BrdU exactly as in a , but were killed earlier and were labelled with EdU 4 and 20 h before death. ( e ) Sections from control (G s α fl/fl) and G s α cKO (Col2-CreERt; G s α fl/fl) mice treated as shown in d were stained with both BrdU and EdU. Double BrdU- and EdU-labelled cells (arrows) were observed in G s α cKO mice but almost never in control mice. ep=epiphyseal bone. Scale bars, 100 μm. Full size image We next examined possible changes in the proliferation and apoptosis of the reserve chondrocytes in the PPR and Gsα cKOs. Since increased proliferation was observed in G s α cKO chondrocytes until final remnant formation ( Figs 2a,e and 3b , Supplementary Fig. 2c and data in text), we tested whether recruitment of stem-like chondrocytes into the proliferative pool was accelerated in G s α-deficient mice. A double BrdU and EdU labelling protocol ( Fig. 5d ) was utilized to address this question. BrdU was used to label slowly replicating chondrocytes, while EdU was used to label chondrocytes that were proliferating just before killing. Indeed, an increased number of double BrdU+EdU-positive cells was observed upon G s α ablation (percent of double BrdU+EdU-positive cells among BrdU-positive cells was 1.7±1 and 13.8±4% in control and G s α cKO mice, respectively, P <0.05 by t -test, n =6; Fig. 5e ), suggesting increased recruitment of stem-like chondrocytes into the proliferative pool. Control experiments showed no cross-reactivity in detection of EdU and BrdU ( Supplementary Fig. 4 ). Interestingly, the number of stem-like chondrocytes recruited into the proliferative pool was not elevated upon ablation of the PPR (1.25±0.1 in control versus 0.7±0.3 double-positive cells per section in PPR cKO mice, P =0.09 by t -test, n =5, see also Fig. 6a,b ). (In this protocol, ( Fig. 6a ), we administered tamoxifen 3–4 days before killing, because changes occur very rapidly in the PPR cKO mice.) However, a clear reduction in the total number of stem-like chondrocytes was observed as early as 3.5 days after PPR ablation (24±2 versus 38±2 BrdU-positive cells/growth plate in control, n =5, P <0.001 by t -test). Analysis of cell death revealed that ablation of the PPR increased the number of apoptotic cells in the reserve zone of the growth plate threefold (4.9±1.0% TUNEL-positive cells in the resting zone of the growth plate in PPR cKO mice versus 1.5±0.4% in control mice, n =5, P <0.05 by t -test). To check whether specifically stem-like chondrocytes were dying upon PPR ablation, we labelled stem-like chondrocytes with BrdU ( Fig. 6a ) and performed double TUNEL plus BrdU detection. Indeed, upon PPR ablation there was a 2.9-fold increase in the number of double BrdU+TUNEL-positive cells (5.8±1.3 double BrdU+TUNEL-positive cells per growth plate versus 2±0.4 in control, n =5, P <0.05 by t -test; Fig. 6c ). No increase in double BrdU+TUNEL-positive cells was observed upon G s α ablation ( Fig. 7 ; 1.8±0.2 in control versus 1.6±0.5 double-positive cells in G s α cKO mice, P =0.7 by t -test, n =5). 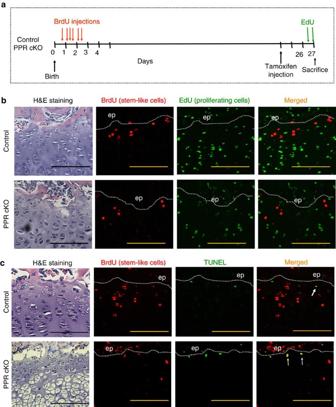Figure 6: Cells of the reserve zone are not recruited into the proliferative pool but undergo apoptosis in PPR cKO mice. (a) Scheme showing BrdU labelling of reserve zone cells (stem-like chondrocytes) and EdU labelling of proliferating chondrocytes in the growth plate of control (PPR fl/fl) and PPR cKO (Col2-CreERt; PPR fl/fl) mice. (b) Sections from control and PPR cKO mice treated as shown inawere stained for both BrdU and EdU. Double BrdU- and EdU-labelled cells were not observed in PPR cKO mice. (c) Sections from control and PPR cKO mice treated as shown inawere stained for both BrdU and simultaneously for apoptosis (TUNEL). Increased number of double TUNEL+BrdU-positive cells (arrows) was observed in PPR cKO mice as compared with control mice. Scale bars, 100 μm. Figure 6: Cells of the reserve zone are not recruited into the proliferative pool but undergo apoptosis in PPR cKO mice. ( a ) Scheme showing BrdU labelling of reserve zone cells (stem-like chondrocytes) and EdU labelling of proliferating chondrocytes in the growth plate of control (PPR fl/fl) and PPR cKO (Col2-CreERt; PPR fl/fl) mice. ( b ) Sections from control and PPR cKO mice treated as shown in a were stained for both BrdU and EdU. Double BrdU- and EdU-labelled cells were not observed in PPR cKO mice. ( c ) Sections from control and PPR cKO mice treated as shown in a were stained for both BrdU and simultaneously for apoptosis (TUNEL). Increased number of double TUNEL+BrdU-positive cells (arrows) was observed in PPR cKO mice as compared with control mice. Scale bars, 100 μm. 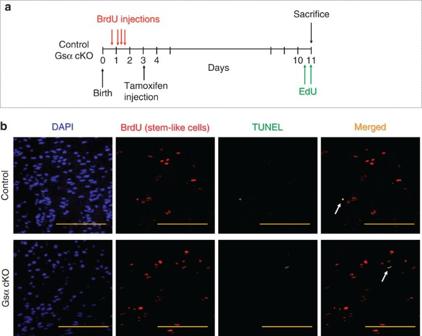Figure 7: Cells of the reserve zone do not undergo apoptosis in Gsα cKO mice. (a) Scheme showing BrdU labelling of reserve zone cells (stem-like chondrocytes) and EdU labelling of proliferating chondrocytes in the growth plate of control (Gsα fl/fl) and Gsα cKO (Col2-CreERt; Gsα fl/fl) mice. (b) Sections from control and Gsα cKO mice shown inawere stained for both BrdU and for a marker of apoptosis (TUNEL). There were no differences in the small number of double TUNEL+BrdU-positive cells (arrows). Scale bars, 100 μm. Full size image Figure 7: Cells of the reserve zone do not undergo apoptosis in G s α cKO mice. ( a ) Scheme showing BrdU labelling of reserve zone cells (stem-like chondrocytes) and EdU labelling of proliferating chondrocytes in the growth plate of control (G s α fl/fl) and G s α cKO (Col2-CreERt; G s α fl/fl) mice. ( b ) Sections from control and G s α cKO mice shown in a were stained for both BrdU and for a marker of apoptosis (TUNEL). There were no differences in the small number of double TUNEL+BrdU-positive cells (arrows). Scale bars, 100 μm. Full size image Thus, stem-like chondrocytes behave differently upon ablation of either G s α or the PPR. Upon ablation of G s α, these cells move into the proliferative pool, whereas, upon ablation of the PPR, they undergo apoptosis at a greatly increased rate. Stem-like chondrocytes need both G s α and G q/11 α signalling We next hypothesized that additional heterotrimeric G-proteins activated by the PPR may contribute to the observed differences in the behaviour of stem-like chondrocytes and remnant formation. To address this question, we surveyed all other G-proteins known to be activated by the PPR in chondrocytes. First, we investigated the role of the extra-large alpha subunit (XLαs), a splice variant of G s α with a different initial coding exon and otherwise identical exons 2–13 used to encode G s α [15] ; XLαs activates adenylate cyclase but also has some actions that differ from those of G s α [8] , [15] . Changes in the growth plate and pattern of BrdU incorporation of mice without both G s α and XLαs were identical to those found in the mice without G s α alone ( Supplementary Fig. 5 ), and remnant formation was observed in the absence of both XLαs and G s α ( Supplementary Fig. 5d ), suggesting no major role for XLαs in the postnatal growth plate when G s α is ablated. Further, ablation of Gα12 and Gα13 utilizing conventional Col2-Cre ( Supplementary Fig. 6 ) caused no changes in the growth plate morphology, level of chondrocyte proliferation, bone length or body weight. Therefore, we conclude that Gα12/13 G-proteins are not required for normal growth plate morphology in postnatal life. A role for the G q/11 α heterotrimeric G-protein family in mediating the action of the PPR was previously analysed in the fetal growth plate, utilizing a ‘knock-in’ mouse expressing only PTH receptors mutated to allow normal G s α activation but no activation of G q/11 α (DSEL mutation) [9] , [16] , [17] . In fetal life, this mutation led to delayed chondrocyte differentiation [9] . Because chondrocytes from the heterozygous DSEL mice (D/+) and wild-type mice indistinguishably activate phospholipase C [9] , we used D/+ mice as a surrogate for WT mice to simplify the mating schemes of these experiments. No growth plate phenotype was observed in postnatal life in DSEL mice as compared with D/+ mice; the overall morphology of the growth plate and the proliferative/apoptotic profiles of stem-like chondrocytes were normal ( Fig. 8a–d and Supplementary Table 1 ). To characterize the role of G q/11 α in stem-like cell behaviour in the absence of G s α, we crossed G s α cKO mice with DSEL mice. Fusion of the growth plate was observed in mice without both G s α and G q/11 α signalling (G s α cKO plus homozygous DSEL mutation of PPR (Col2-CreERt; G s α fl/fl; PPR D/D). In contrast, G s α cKO mice heterozygous for the DSEL mutation (PPR +/D) retained a remnant ( Fig. 9a ). Small cartilage remnants could occasionally be observed in the homozygous D/D mutants missing G s α (two mice out of eight examined; one such remnant is shown in Fig. 9b ). At an early time point (11 days after Tam administration), clear acceleration of growth plate fusion was observed in the absence of both G s α and G q/11 α (area of the growth plate 99,700±10,500 pixels in Col2-CreERt; G s α fl/fl; D/+ versus 47,900±7,950 pixels in Col2-CreERt; G s α fl/fl; D/D, P <0.05 by t -test). As with ablation of the PPR ( Supplementary Fig. 1e ), ablation of both G s α and G q/11 α signalling abrogated chondrocyte proliferation ( Fig. 9c ), while this was not observed upon ablation of G s α alone ( Fig. 2e and Supplementary Fig. 2a,c ). Furthermore, ablation of both G s α and G q/11 α elevated apoptosis in the resting zone (1.5±0.3% of round stem-like cells are TUNEL-positive cells in G s α fl/fl; D/D mice versus 7.3±1.0% in Col2-CreERt; G s α fl/fl; D/D mice, n =8, P <0.001 by t -test; see also Fig. 9d ). This result was similar to the effect observed upon ablation of PPR ( Fig. 6c ), but not with G s α alone ( Figs 2b and 7b ). Further, the number of cells positive for cleaved caspase-3 was increased 3.9-folds in the resting zone of Col2-CreERt; G s α fl/fl; D/D mice as compared with G s α fl/fl; D/D mice (1.74±0.3 versus 0.45±0.15%, P <0.05 by t -test, n =4, Fig. 8e ). To directly test whether these dying cells are stem-like chondrocytes, we labelled slowly replicating cells with multiple BrdU injections (using the same protocol as in Fig. 7a ) and performed double TUNEL plus BrdU detection. Indeed, a 3.4-fold increase in the number of double BrdU+TUNEL-positive cells was observed upon substitution of both copies of PPR with the DSEL mutant in the absence of G s α (2.0±0.5 double BrdU+TUNEL-positive cells in Col2-CreERt; G s α fl/fl; D/+ versus 6.8±0.5 in Col2-CreERt; G s α fl/fl; D/D, n =5, P <0.001 by t -test; Fig. 9e ). 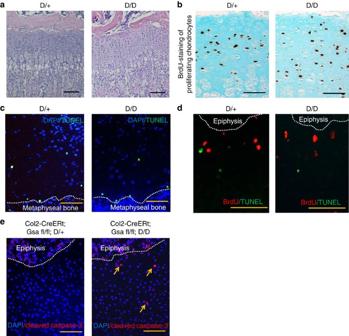Figure 8: Characterization of DSEL mice alone and in combination with Gsα KO. (a–d) DSEL mice9. No changes were observed in the growth plate height (a), BrdU incorporation (b), apoptosis (c) and BrdU-labelled stem-like cells co-visualized with TUNEL-positive cells (d, experimental details are the same as forFig. 7a) between mice with one copy of mutated PTH receptor (DSEL mutation, D/+) and two copies of the mutated receptor (D/D). (e) In mice with inactivated Gsα in their growth plate, the DSEL mutation of two copies of the PTH receptor increased the number of cells positive for cleaved caspase-3 as compared with those in which only one copy of the PTH receptor was mutated. Tamoxifen was injected at 3 days of age and mice were analysed 9 days later. Scale bars, 100 μm. Figure 8: Characterization of DSEL mice alone and in combination with G s α KO. ( a – d ) DSEL mice [9] . No changes were observed in the growth plate height ( a ), BrdU incorporation ( b ), apoptosis ( c ) and BrdU-labelled stem-like cells co-visualized with TUNEL-positive cells ( d , experimental details are the same as for Fig. 7a ) between mice with one copy of mutated PTH receptor (DSEL mutation, D/+) and two copies of the mutated receptor (D/D). ( e ) In mice with inactivated G s α in their growth plate, the DSEL mutation of two copies of the PTH receptor increased the number of cells positive for cleaved caspase-3 as compared with those in which only one copy of the PTH receptor was mutated. Tamoxifen was injected at 3 days of age and mice were analysed 9 days later. Scale bars, 100 μm. 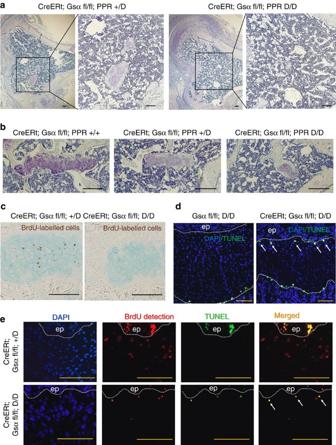Figure 9: Simultaneous ablation of Gsα from chondrocytes and Gq/11α signalling from the PPR. A gene (D) encoding a PTH/PTHrP receptor mutated so that it cannot activate Gq/11 G-proteins9was introduced into Col2-CreERt; Gsα fl/fl mice. Tamoxifen was administrated at 3 days of age. Mice without Gsα signalling (Col2-CreERt; Gsα fl/fl) and with one or two copies of mutated PPR (D/+ or D/D) were compared. (a,b) One month after tamoxifen injection, fusion of the growth plate was observed in all tibias (a) in the mice lacking Gsα having mutated PPR, whereas small remnant can still be observed in some femurs (two out of eight animals analysed,b), genotypes as indicated. (c) Cessation of chondrocyte proliferation (assessed as BrdU incorporation 11 days after tamoxifen administration) and (d) elevation of ectopic apoptosis in the resting zone (assessed by TUNEL 9 days after tamoxifen administration, arrows). (e) Stem-like chondrocytes were labelled with BrdU as inFig. 7aand stained for both BrdU and for apoptosis (TUNEL). Dotted lines depict growth plates. ep=epiphyseal bone. Scale bars, 100 μm. Full size image Figure 9: Simultaneous ablation of Gsα from chondrocytes and G q/11 α signalling from the PPR. A gene (D) encoding a PTH/PTHrP receptor mutated so that it cannot activate Gq/11 G-proteins [9] was introduced into Col2-CreERt; G s α fl/fl mice. Tamoxifen was administrated at 3 days of age. Mice without G s α signalling (Col2-CreERt; G s α fl/fl) and with one or two copies of mutated PPR (D/+ or D/D) were compared. ( a , b ) One month after tamoxifen injection, fusion of the growth plate was observed in all tibias ( a ) in the mice lacking G s α having mutated PPR, whereas small remnant can still be observed in some femurs (two out of eight animals analysed, b ), genotypes as indicated. ( c ) Cessation of chondrocyte proliferation (assessed as BrdU incorporation 11 days after tamoxifen administration) and ( d ) elevation of ectopic apoptosis in the resting zone (assessed by TUNEL 9 days after tamoxifen administration, arrows). ( e ) Stem-like chondrocytes were labelled with BrdU as in Fig. 7a and stained for both BrdU and for apoptosis (TUNEL). Dotted lines depict growth plates. ep=epiphyseal bone. Scale bars, 100 μm. Full size image The marked decrease in chondrocyte proliferation in the absence of both G s α and Gq/11 signalling, when the absence of either signalling pathway alone did not decrease chondrocyte proliferation, is surprising. Because cyclin D1 participates in regulating cell proliferation and is known to be regulated in chondrocytes by PTHrP [18] , we determined the levels of cyclin D1 expression in the growth plates of mice with single and double pathway ablation. Inactivation of Gq/11 signalling did not affect levels of cyclin D1 in chondrocytes in the presence of intact G s α signalling, when we scored the percentage of cyclin D1 immuno-reactive cells in the flat cell layer (26±4% in D/+ versus 24±4% of cyclin D1 positive cells in D/D mice, P =0.8 by t -test, n =3, see also Fig. 10a,b ), but inactivation of Gq/11 signalling did lower cyclin D1 with reduced G s α signalling (26±2% in Col2-CreERt; Gsa fl/+; D/+ versus 16±3% in Col2-CreERt; Gsa fl/+; D/D, P <0.05 by t -test, n =3, see also Fig. 10c,d ) or in the absence of G s α signalling (9±2% in Col2-CreERt; Gsa fl/fl; D/+ versus 1±1% in Col2-CreERt; Gsa fl/fl; D/D, P <0.05 by t -test, n =5, see also Fig. 10e–h ). Thus, cyclin D1 may be one of the crucial gene targets that explain the contrasting proliferation phenotypes of the Gsα and PPR cKO growth plates. 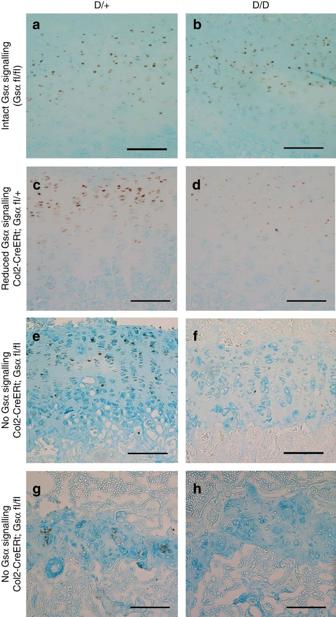Figure 10: Levels of cyclin D1 are regulated by both Gsα and Gq/11 signalling from PTH receptor. Levels of cyclin D1 were compared between mice with one copy of mutated PTH receptor (DSEL mutation, D/+) and two copies of the mutated receptor (D/D) in the presence or absence of Gsα. No changes were observed in the levels of cyclin D1 in the presence of intact Gsα signalling and impaired Gq/11 signalling (a,b). Inactivation of Gq/11 signalling in the absence of one allele of Gsα decreases levels of cyclin D1 (c,d) as well as inactivation of Gq/11 in the absence of both allels of Gsα (e–h). Tamoxifen was injected at 3 days of age and levels of cyclin D1 were analysed by immonohistochemistry 12 days later (a–f) or 15 days later (g,h). Scale bars, 100 μm. Figure 10: Levels of cyclin D1 are regulated by both G s α and Gq/11 signalling from PTH receptor. Levels of cyclin D1 were compared between mice with one copy of mutated PTH receptor (DSEL mutation, D/+) and two copies of the mutated receptor (D/D) in the presence or absence of G s α. No changes were observed in the levels of cyclin D1 in the presence of intact G s α signalling and impaired Gq/11 signalling ( a , b ). Inactivation of Gq/11 signalling in the absence of one allele of G s α decreases levels of cyclin D1 ( c , d ) as well as inactivation of Gq/11 in the absence of both allels of G s α ( e – h ). Tamoxifen was injected at 3 days of age and levels of cyclin D1 were analysed by immonohistochemistry 12 days later ( a – f ) or 15 days later ( g , h ). Scale bars, 100 μm. Full size image Thus, we conclude that, while G s α is the predominant mediator of the effects of PTHrP on chondrocyte maturation, both G s α and G q/11 α synergize to prevent growth plate disappearance, preserve chondrocyte proliferation and protect stem-like chondrocytes from cell death (observed phenotypes are summarized in Supplementary Table 2 ). Here we found that ablation of G s α drives stem-like chondrocytes to proliferate, whereas ablation of the PPR leads to their apoptotic elimination. The diverse actions of the PPR and its second message systems may combine both cell-autonomous actions of these pathways on chondrocytes, as well as more complicated actions on signalling between cells in the growth plate. For example, elevated Ihh levels are observed in both PPR [10] - and G s α− ( Fig. 2d ) deficient growth plates. The increase in Ihh levels might trigger different responses in cells deficient for either PPR (response–cell death) or G s α (response–recruitment into the proliferative pool). In wild-type mice, Ihh stimulates conversion of round cells into flat proliferating chondrocytes in fetal life [19] . Ablation of G s α leads to transformation of the growth plate into a so-called cartilage remnant, disorganized epiphyseal cartilage with cells paused in the middle of their differentiation path. In contrast, ablation of the PPR [10] ( Fig. 1e ) leads to closure of the growth plate. It is reasonable to speculate that differing properties of stem-like and/or flat cell chondrocytes in these two models contribute to the difference. In the absence of the PPR, stem-like cells have increased apoptosis, while in the absence of G s α they start proliferating. This increased conversion of stem-like chondrocytes into proliferative chondrocytes in G s α cKO mice ( Supplementary Fig. S2c ) may contribute to the persistent proliferation of chondrocytes in these mice observed 9 and 14 days after tamoxifen administration. Furthermore, flat cells have decreased proliferation in PPR cKO mice. Both movement of stem-like cells into the proliferative pool and elevated proliferation of these cells should lead to a larger number of chondrocytes entering the prehypertrophic pool in G s α cKO mice, thereby contributing to remnant formation. Nevertheless, we cannot explain why this larger group of chondrocytes cannot further differentiate, die and otherwise be resorbed. One possible speculation could be that disorganization of the growth plate observed from day 14 onwards interferes with signals needed for proper chondrocyte terminal differentiation, such as Mef2C levels or BMP signalling. Alternatively, encapsulation of the remnant into epiphyseal bone might physically separate the remnant from cells capable of resorbing cartilage. The striking differences between PPR and G s α cKO growth plate phenotypes mandate that other signalling pathways downstream of the PPR, in addition to G s α, must mediate the receptor’s actions. To identify them, we have genetically screened all G-proteins reported to be activated by the PPR. Among those, activation of the G q/11 α by the PPR contributes to the full action of the PPR. Indeed, ablation of G s α and G q/11 α signalling closely mimics ablation of the PPR. Thus, our data suggest that activation of both G s α and G q/11 α by the PPR is required for stem-like chondrocytes to stay in the quiescent phase. Indeed, synergism between the actions of PKA (G s α pathway) and PKC (G q/11 α pathway) is widely described [20] , [21] , [22] , [23] . Here we show such synergism in the regulation of cyclin D1 levels in columnar growth plate chondrocytes ( Fig. 10 ). Interestingly, ablation of the PPR leads to ectopic apoptosis in the resting zone only in postnatal, but not in the fetal growth plate [10] , suggesting different mechanisms related to regulation of stem-like chondrocytes in fetal and postnatal growth plates. In conclusion, our data suggest that PPR signalling in the postnatal growth plate is responsible for keeping stem-like chondrocytes in a quiescent state and that activation of downstream G s α and G q/11 α signalling pathways determines the fate of these cells. Simultaneous activation of both pathways keeps chondrocytes in a quiescent state; activation of the G q/11 α without activation of G s α stimulates cells to enter the cell cycle, whereas inactivation of both pathways eliminates these cells through programmed cell death. Mice A transgenic mouse strain harbouring Collagen 2-driven Cre fused with a mutated oestrogen receptor ligand-binding domain (Col2-CreERt) was used to induce ablation of floxed genes in cartilage upon tamoxifen administration. Mice with floxed exon 1 of the GNAS1 gene were utilized for G s α inactivation. Mice with floxed essential exon E1 of the PPR gene were utilized for PPR inactivation. All mice have been previously described: mice with floxed exon 1 of Gnas gene (G s α fl/fl mice) [11] , mice with floxed exon E1 of the PTH receptor (PPR fl/fl mice) [24] , mice with a clustered point mutation in the PTH receptor leading to selective inability to activate the G q/11 α pathway (DSEL mice) [9] , mice with exon 2 of the Gnas gene disrupted [15] , mice with inactivated Gnα12 (ref. 25 ), mice with floxed exon 2 of Gnα13 (ref. 26 ), transgenic mice expressing Cre linked to a mutated ligand-binding domain of oestrogen receptor α that can bind tamoxifen but not β-oestradiol under the control of the collagen 2 α1 promoter (Col2-CreERt mice) [27] and transgenic mice expressing Cre under the control of the collagen 2 α1 promoter (Col2-Cre mice) [24] . Rosa reporter mice, with cre-dependent β galactosidase expression, were as described [28] . Primers utilized for genotyping are listed in Supplementary Table 3 . The following genetic backgrounds were used: PPR mice were backcrossed onto a C57/Bl6 background for six generations. G s α mice were on mixed background ( Figs 1 , 2 , 3a–e and 4 ), six generations backcrossed onto a CD-1 background ( Fig. 3f , Supplementary Fig. 5 ) and six generations backcrossed onto a C57/Bl6 background ( Figs 5 and 7 , Supplementary Fig. 3b,c ). DSEL mice were backcrossed onto a C57/Bl6 background for more than 10 generations. Gnas exon 2 mice were backcrossed onto a CD-1 background for six generations. Gα12 and Gα13 were backcrossed onto a CD-1 background for five generations. The study was approved by the Institutional Animal Care and Use Committee of the Massachusetts General Hospital and by the Local Ethics Committee at Karolinska Institutet, Stockholm, Sweden. Details for XLαs breeding To address the role of XLαs in the growth plate in vivo and its contribution to remnant formation in G s α cKO mice, we employed mice with disrupted exon 2 of GNAS1 (Ex2-Neo-G s α), an exon required for expression of both G s α and XLαs [15] . Ex2-Neo-G s α heterozygotes survive and are fertile. Taking advantage of the fact that in chondrocytes XLαs is expressed from only the paternal allele [8] , we crossed Ex2-Neo-G s α males with Col2-CreERt; G s α fl/fl females. Progeny were injected with tamoxifen at 3 days of age, and pups with Col2-CreERt, GNAS1 floxed in exon 1 (inherited from the mother) and GNAS1 with exon 2 disrupted (exon2-Neo, inherited from the father) were considered null for both XLαs and G s α. Finally, we crossed males with one allele of GNAS1 disrupted by insertion of a neo cassette into exon 2 and a second allele with floxed exon1 (Ex2-Neo-G s α/G s α-fl) with Col2-CreERt; G s α fl/fl females, injected pups with tamoxifen at 3 days of age and evaluated remnant formation 1 month later. Details for Gα12 and Gα13 breeding To address the role of Gα12 and Gα13 in bone growth, we crossed Gα12-deficient mice (G12−/−) with Gα13-floxed mice (G13fl/fl) and then with Col2-CreERt transgenic mice. Mice of both sexes were injected 0.5 mg tamoxifen at 3 days of age. The following genotypes were compared in different combinations: G12+/−;G13fl/+, G12−/−;G13fl/+, G12−/−;G13fl/fl, Col2-CreERt;G12+/−;G13fl/+, Col2-CreERt;G12−/−;G13fl/+, Col2-CreERt;G12+/−;G13fl/fl, Col2-CreERt;G12−/−;G13fl/fl. At least three animals of each genotype were analysed. The same breeding strategy was employed utilizing conventional Col2-Cre. Genotyping and PCR Genotyping of mice was performed by PCR as described in the original publications, as well as in related articles (see list of original primers used for routine genotyping in Supplementary Table 3 ) except that for Gnas exon 2 mice. For these mice, the primers were redesigned not to interfere with genotyping of G s α mice floxed in exon 1. For genotyping of neo-disrupted exon 2 of Gnas , the combination of the following three primers was used: forward-1 5′-TTGTTTTTCACTGCGTCGTC-3′; reverse-1 5′-CTTCCATTTGTCACGTCCTG-3′; and reverse-2 5′-CCTTCAAACGTCCTGTCTCC-3′ with a 435-bp fragment from the neo-cassette-disrupted allele and a 303-bp fragment from the WT allele of the Gnas gene. For detection of G s α recombination, primers utilized for genotyping (5′-GAGAGCGAGAGGAAGACAGC-3′ and 5′-TCGGGCCTCTGGCGGAGCTT-3′, 390 bp floxed allele and 330 bp WT allele) were combined with 5′-AGCCCTACTCTGTCGCAGTC-3′, giving a 250-bp PCR product upon recombination (see Supplementary Fig. 7 ). Tamoxifen administration Tam (Sigma) was dissolved in corn oil (Sigma) at a concentration of 10 mg ml –1 . Three-day-old mice of both sexes were injected i.p. 0.5 mg Tam per each mouse if not otherwise indicated. X-gal staining β-galactosidase activity was evaluated using X-gal staining, which was performed on either entire bone or unfixed frozen sections using the ‘Stain for Beta-Gal Expression In Tissue’ and ‘Stain for Beta-Gal Expression In Situ’ kits (Millipore) following the manufacturer’s protocol. Skeletal preparation Alizarin red and Alcian blue staining were performed using a modification of McLeod’s method [29] . Bones were dissected out, fixed in 95% ethanol overnight and stained in alcian blue solution (0.015% alcian blue (Sigma) in 80% ethanol and 20% acetic acid) overnight. Thereafter, bones were washed in 95% ethanol a few times and transferred to 2% KOH for removal of the remaining soft tissue followed by staining in alizarin solution (0.005% alizarin sodium sulphate (Sigma) in 1%KOH) overnight. Next, bones were cleared in 1%KOH in 20% glycerol for at least 2 days and stored in 1:1 mixture of glycerol with 95% ethanol until images captured. Tissue preparation For all techniques outlined below, tissues were prepared as following. Mice were dissected, bones were fixed in 4% (vol/vol) paraformaldehyde/PBS, decalcified in 10% (wt/vol) EDTA, processed, embedded in paraffin, and 5-μm-thick sections were obtained. Distal femur and both proximal and distal tibia growth plates were analysed. In all images the proximal tibia growth plate is shown if not otherwise indicated. Histological analysis For histological analysis, sections were stained with hematoxylin and eosin (H&E). Images were captured using a Nikon Eclipse E800 light microscope and analysed by using ImageJ software (NIH, Bethesda). The height of the growth plate was calculated as an average of 30 measurements, and at least two sections for every animal were analysed. At the columnar to hypertrophic transition, only cells with height lower than 7 μm were considered as columnar chondrocytes. The height of the terminal hypertrophic chondrocytes, the cell in the last intact lacuna, was measured in 24 different columns per growth plate and averaged. For linear measurements, pixels were converted into micrometers using images of a calibration scale. Data for remnant area are presented in pixels, and all pictures analysed were taken simultaneously with the same magnification and resolution. In situ hybridization In situ hybridization was performed as described elsewhere [8] , [24] . Specifically, sections were rehydrated, post-fixed in 4% PFA for 5 min, treated with 2 μg ml –1 of Proteinase K for 10 min, acetylated, washed and air-dried. Hybridization was carried out at 60 °C overnight. Riboprobes were DIG-labelled and upon hybridization detected according to a Roche Applied Science Inc protocol, utilizing an ant-DIG alkaline phosphatase-conjugated antibody (Roche). For fluorescent probe visualization, an anti-DIG antibody conjugated with peroxidase (Roche) was used, followed by signal amplification with a TSA-biotin system (Perkin Elmer) and visualization with streptavidin conjugated with Alexa-594 (Invitrogen). The following probes were used: probes for mouse type X collagen (nucleotides 903–2215, GenBank accession no. X65121, subcloned in pBlueScript, provided by Bjorn Olsen, Harvard Medical Scool), Patched 1 (4.3 kb mouse cDNA subcloned in pBS, provided by Ron L Johnson, Stanford University), Ihh (nucleotides 1–557 of mouse Ihh cDNA subcloned in pBS,) and osteopontin (nucleotides 157–1144; GenBank accession no. X14882, provided by Ernestina Schipani, University of Michigan). Probes for rat G s α (full-length cDNA) and rat XLαs (nucleotides 380–1154, Gen- Bank accession no. X84047) were provided by Dr Murat Bastepe (Massachusetts General Hospital and Harvard Medical School). Apoptosis assay Apoptotic cells were identified using a TUNEL-based in situ cell death detection kit (Roche Diagnostics, cat. # 11684795910). After treatment with 10 μg ml –1 proteinase K for 30 min at 37 °C, sections were incubated with the TUNEL reaction mixture for 1.5 h at 37 °C, rinsed and mounted with Vectashield containing DAPI (Vector Laboratories, cat. # H-1200). Immunohistochemistry Immunohistochemistry was performed as described elsewhere [10] . Specifically, sections were rehydrated and antigen retrieval was performed in citrate buffer. Endogenous peroxidase was blocked by incubation in 3% H 2 O 2 for 10 min, and blocking was accomplished with 3% horse serum for 1 h. Primary antibodies were incubated overnight at 4 °C, and corresponding secondary biotinylated antibody was subsequently incubated for 1–2 h at room temperature. Visualization was accomplished by incubation with streptavidin conjugated with either fluorochrome or peroxidase. Primary antibodies against G s α (K-20, 1:100 dilution, Santa Cruz Biotechnology), Gα13 (A-20, 1:200 dilution, Santa Cruz Biotechnology), cleaved caspase 3 (1:50 dilution, Cell Signaling), Mef2c (1:500 dilution, Sigma), protein kinase A (PKA) substrate (1:100 dilution, Cell Signaling), cyclin D1 (1:50 dilution, Cell Signaling), phospho-SMAD1/5 (1:50 dilution, Cell Signaling), Ki67 (1:50 dilution, Dako) or Sox9 (1:1,000 dilution, Sigma Aldrich) and the TSA biotin system kit (Perkin Elmer, cat. # NEL700A001KT) were used as recommended by the manufacturers. Immunoreactive proteins were visualized using the avidin-biotin-peroxidase complex, followed by incubation with the DAB substrate kit (Vector Laboratories) or streptavidin conjugated with Alexa-594 (Invitrogen) for fluorescent detection. Alcian Blue was used for counterstaining of non-fluorescent images. Non-immune rabbit IgG were used as a negative control for both K-20 and A-20 antibodies and showed no staining. Corresponding blocking peptide (Cell Signaling) was used for PKA substrate antibodies and showed no staining. Labelling index for CyclinD1 immuno-positive cells was calculated as a number of immuno-positive chondrocytes divided by the total number of chondrocytes in the area in which CyclinD1-positive cells were detected. BrdU labelling and detection For BrdU labelling, BrdU was injected to mice (100 μg g –1 i.p.) 2–4 h before killing if not otherwise specified. BrdU was detected using the BrdU staining kit (Zymed). For fluorescent visualization, streptavidin conjugated with peroxidase was substituted by streptavidin conjugated with Alexa 594 (Invitrogen) followed by washing and mounting with Vectashield containing DAPI (Vector Laboratories). The BrdU labelling index was calculated as the ratio of BrdU-positive nuclei over total nuclei in each region of the growth plate (percent of positive cells). Alcian Blue and 50 times-diluted Eosin stainings were used for counterstaining of non-fluorescent images. Double EdU plus BrdU labelling and detection For labelling stem-like chondrocytes, BrdU was injected i.p. (20 μg g –1 ) every 6–8 h during the first 2 days of life, and mice were killed at indicated time points. EdU (50 μg g –1 ) was injected 24 and 4 h before death. BrdU was detected using an anti-BrdU antibody (Sigma-Aldrich) followed by a secondary biotinylated antibody and streptavidin conjugated with Alexa-594 (Invitrogen). Thereafter, sections were subjected to EdU detection that was performed according to the manufacture’s instructions (Invitrogen). Double TUNEL plus BrdU detection Apoptotic cells were visualized by TUNEL as described above, followed by detection of BrdU-positive cells as described above for ‘Double EdU plus BrdU labelling and detection’. Control experiments revealed less than 3% of false-negative TUNEL-positive cells after double detection versus single TUNEL detection. Statistical methods All data are expressed as mean±s.e.m. when appropriate. The differences between groups were evaluated using an unpaired t -test. N stands for number of animals analysed; several sections were analysed for every mouse. How to cite this article: Chagin, A. S. et al. G-protein stimulatory subunit alpha and Gq/11α G-proteins are both required to maintain quiescent stem-like chondrocytes. Nat. Commun. 5:3673 doi: 10.1038/ncomms4673 (2014).